Boosting electrocatalytic CO2–to–ethanol production via asymmetric C–C coupling Electroreduction of carbon dioxide (CO 2 ) into multicarbon products provides possibility of large-scale chemicals production and is therefore of significant research and commercial interest. However, the production efficiency for ethanol (EtOH), a significant chemical feedstock, is impractically low because of limited selectivity, especially under high current operation. Here we report a new silver–modified copper–oxide catalyst (dCu 2 O/Ag 2.3% ) that exhibits a significant Faradaic efficiency of 40.8% and energy efficiency of 22.3% for boosted EtOH production. Importantly, it achieves CO 2 –to–ethanol conversion under high current operation with partial current density of 326.4 mA cm −2 at −0.87 V vs reversible hydrogen electrode to rank highly significantly amongst reported Cu–based catalysts. Based on in situ spectra studies we show that significantly boosted production results from tailored introduction of Ag to optimize the coordinated number and oxide state of surface Cu sites, in which the * CO adsorption is steered as both atop and bridge configuration to trigger asymmetric C–C coupling for stablization of EtOH intermediates. Electroreduction of carbon dioxide (CO 2 ) to high-value chemicals and fuels is seen to be practically promising for the utilization of renewable electricity and mitigation of CO 2 emissions, which has emerged as a frontier in energy conversion and carbon neutrality [1] , [2] , [3] . During the CO 2 reduction reaction (CO 2 RR), the applied electrical energy is converted to stored chemical energy via reorganizing the molecular bonds in CO 2 and water to generate products with one (C 1 ), or two or more (C 2+ ) carbon atoms, under the effect of catalysts [4] , [5] , [6] . Most metal catalysts such as gold (Au), silver (Ag), tin (Sn), and lead (Pb) generate a mix of C 1 products [7] , [8] , whilst only Cu-based catalysts transform CO 2 toward C 2+ products via coupling the adsorbed * CO intermediates [9] , [10] , [11] . Amongst the various C 2+ products formed on Cu catalysts, EtOH is important as the liquid fuel because of its wide application and high-energy-density and because it provides the possibility of long-term, large-scale and seasonal energy storage, and convenient transport [3] , [12] . The production of EtOH with high current density and Faradaic efficiency (FE) via Cu-based catalysts is significant to advancing CO 2 RR as a renewable chemical feedstock [2] , [3] , [13] . During CO 2 RR, EtOH and ethylene (C 2 H 4 ) are both 12-electron reduced products, and share the initial intermediates * HCCOH. Given the more saturated structure of EtOH compared with that for C 2 H 4 , the next-intermediates for EtOH are more difficult to stabilize on a pure Cu surface compared with C 2 H 4 . The production of EtOH via C–O bond-reserving of * HCCOH will therefore have chemical difficulty in competing with C 2 H 4 generation. This typically results in the EtOH production in the range of 2–3 times less than that for C 2 H 4 on Cu-based catalyst [3] , [11] , [12] , [13] , [14] . To boost EtOH production, research interest has concentrated on optimal re-design of Cu-based catalysts [5] , [6] , [15] , [16] , [17] , [18] , [19] , [20] , [21] , [22] . Strategies including, control of morphology and facet [16] , [17] , vacancy steering [18] , dopant and modification engineering [19] , [20] , and defects control [21] , [22] have been reported. Among these, the modification of Cu with other CO 2- –active metals to form Cu-based bimetallic is reported as practically attractive [15] , [23] , [24] , [25] , [26] , [27] , [28] . For example, Jaramillo et al. reported Cu–Au bimetallic catalysts with boosted selectivity for CO 2 RR to EtOH, and a synergistic catalytic pathway with CO–tandem mechanism was proposed that CO was first generated on Au, desorbed and migrated to near Cu active sites where C–C coupling to EtOH was conducted [24] . Zheng et al. reported a boosted EtOH selectivity in a Cu 3 Ag 1 bimetallic catalyst with electron-deficient Cu sites via promoting adsorption of key intermediates [25] . Clark et al. hypothesized that the boosted EtOH selectivity results from Ag-induced strain effects of Cu surfaces that modulate EtOH production and suppresses the hydrogen evolution reaction (HER) [26] . Despite significant progress, the advances of reported bimetallic catalysts for FE of EtOH (FE EtOH ) remain limited, especially the production and output efficiency for EtOH is far from the current target for practical application [29] , [30] , [31] , [32] , [33] , [34] , [35] , [36] , [37] , [38] (i.e., partial current density > 300 mA cm −2 and half-cell cathodic energy efficiencies (EE HC ) > 20%). In addition, the key impact of modified components on intrinsic kinetics of reported Cu-based bimetallic catalysts for CO 2 RR at high conversion rates is unclear, which significantly hinders understanding of the mechanism and catalyst design [3] , [14] . Taken together, there is a need therefore for more efficient catalysts and an improved understanding of the mechanism for CO 2 RR to practically boost EtOH under commercial current densities. Here, through modifying Ag onto cubic Cu 2 O and activating under CO 2 RR, we investigated derived CuAg bimetallics (dCu 2 O/Ag) with controlled morphology, phase, and composition for CO 2 RR at high current operation. In contrast to the Cu 2 O and Au-modified Cu 2 O derivatives which favor the conversion of CO 2 to C 2 H 4 and CO, respectively, the optimal dCu 2 O/Ag 2.3% exhibited an asymmetric C–C coupling to stabilize reaction intermediates for boosted EtOH production under high current density. The as-obtained dCu 2 O/Ag 2.3% exhibits FE and EE HC for EtOH of, 40.8% and 22.4%, respectively. We show in a direct comparison with reported catalysts that it has the greatest reported partial EtOH current density with 326.4 mA cm −2 . In situ studies confirm that the redispersion of Ag into Cu significantly optimizes the coordinated number and oxide state of Cu. In this way, the * CO binding strength is altered to form a blended adsorption configuration, that triggers asymmetric C–C coupling for stabilization of EtOH intermediates, and results in boosted EtOH production. This work constructs an efficient catalyst for CO 2 RR with high EtOH selectivity at commercially relevant current densities, and provides guidance for designing catalysts with tailored selectivity in multi-electron reactions. Catalyst preparation and characterization Pristine Ag-modified Cu 2 O nanocubes (Cu 2 O/Ag NCs) were prepared by a one-pot seed-medium method in which Cu 2 O NCs were achieved via reduction of Cu(OH) 2 at room temperature (RT, 25 °C) with ascorbic acid (AA) as a reducing agent, followed by the addition of AgNO 3 . Because of the appropriate lattice spacing match, the added AgNO 3 rapidly nucleates and grows due to the effect of AA to deposit ‘small’ Ag nanoparticles (Ag NPs) on Cu 2 O NCs surface (Fig. 1a ). Transmission electron microscopy (TEM) images reveal that the Cu 2 O/Ag NCs exhibit heterostructure that Ag NPs sporadically adorn the Cu 2 O surface (Fig. 1b and Supplementary Fig. 1a ), in comparison to Cu 2 O NCs with cubic morphology and a side length of ~45 nm (Supplementary Fig. 2 ). X-ray photoelectron spectroscopy (XPS) and scanning electron microscopy energy-dispersive X-ray spectroscopy (SEM-EDS) confirm that the Ag NPs in Cu 2 O/Ag NCs are metallic, with the content controlled to 2.3% (Fig. 1c and Supplementary Fig. 1b ). High-resolution TEM (HRTEM) image highlights the interplanar spacing of the lattice fringes for Cu 2 O NCs and Ag NPs regions to be 0.214 nm and 0.236 nm in Cu 2 O/Ag 2.3% NCs. This finding is consistent with the Cu 2 O (200) plane and Ag (111) plane, respectively (Fig. 1d ). Powder X-ray diffraction (XRD) was carried out to confirm the phase of Cu 2 O/Ag NCs. It was found that Cu 2 O/Ag NCs exhibit the same peak as for Cu 2 O NCs which is attributed to the low Ag NPs content (Fig. 1e ). In addition, the EDX mapping images for Cu 2 O/Ag 2.3% NCs also display an apparent element separation between Ag NPs and Cu 2 O NCs, (Fig. 1f ). XPS assesses the surface properties of catalysts. The peaks at 951.8 and 931.8 eV for Cu 2 O NCs are ascribed to, Cu 2p 1/2 and 2p 3/2 , respectively, confirming the presence of Cu(I) in Cu 2 O NCs (Fig. 1g ) [39] . Following Ag modification, two shoulder peaks for Cu(II) were apparent in the XPS spectra, demonstrating that electrons transfer from Cu 2 O to Ag. This finding is validated via the Auger electron spectroscopy (AES) for Cu LMM in which the peaks for Cu 2 O/Ag 2.3% NCs downshifts to a lower kinetic energy compared with those for Cu 2 O NCs (Supplementary Fig. 3 ). These findings indicate that an Ag/Cu 2 O heterostructure with altered electron structure for Cu 2 O was reached with Cu 2 O/Ag 2.3% NCs. Fig. 1: Structural characterization of Cu 2 O/Ag NCs. a Schematic for preparation of Cu 2 O/Ag NCs. b TEM image, c Ag 3d XPS curve, d HRTEM images and f EDS elemental mapping images of Cu 2 O/Ag 2.3% NCs. e XRD patterns and g Cu 2p XPS curves for Cu 2 O and Cu 2 O/Ag 2.3% NCs. Scale bars, 10 nm in ( b ), 1 nm in ( d ), and 100 nm in ( f ). White-color, orange and azure spheres in the model represent O, Cu, and Ag atoms, respectively. Full size image Catalyst evolution under CO 2 RR Given the reported evolution of Cu-based catalysts under high current CO 2 RR [36] , activation and in situ characterization was therefore conducted for Cu 2 O/Ag 2.3% NCs to determine the actual state of the catalyst during CO 2 RR. A flow cell with gas diffusion electrode (GDE) was especially designed as a reactor for a high current test (Supplementary Fig. 4 ). As a basis for a detailed comparison, Cu 2 O NCs and Au-modified Cu 2 O NCs (Cu 2 O/Au 2.3% NCs) with similar morphology, composition, and structure to Cu 2 O/Ag 2.3% NCs were synthesized and assessed (Supplementary Fig. 5 ). The catalysts were deposited onto the GDE via spray-coating of the configured ink (details in Supplementary Methods). Activation was controlled by electroreduction of the parent material under CO 2 RR at a current density of 200 mA cm −2 in 1 M KOH for 30 min. The derived Cu-based catalysts obtained following activation supported on the GDE, denoted as dCu 2 O, dCu 2 O/Ag, and dCu 2 O/Au, were subjected to additional characterization. High-angle annular dark-field scanning TEM (HAADF STEM) and SEM images confirm that following activation the original cubic morphology and surface deposited NPs are visually less pronounced, and that instead, ragged surface and hollow structures formed in dCu 2 O/Ag 2.3% and dCu 2 O/Au 2.3% (Fig. 2a and Supplementary Figs. 6 and 7a ). Concomitantly, the original surface phase separation between deposited metal and Cu is lost following activation as is confirmed in EDS mapping images (Fig. 2a , Supplementary Fig. 7b ). The lattice space for dCu 2 O/Ag 2.3% was altered to 0.210 nm following activation, a value near to the Cu (111) facet (Fig. 2b ). Ex situ XRD patterns reveal that the diffraction peaks for Cu 2 O for all catalysts are decreased significantly whilst the diffraction peaks for Cu became dominant. This finding demonstrates that all catalysts are transformed to mainly metallic Cu following activation (Supplementary Fig. 8 ). Compared with dCu 2 O, the XRD peaks of Cu (111) for dCu 2 O/Ag 2.3% and dCu 2 O/Au 2.3% exhibit a meaningful, slight shift to a higher degree to underscore that the original Cu 2 O/metal heterostructures are evolved into the bimetallic alloy following activation (Fig. 2c ). Fig. 2: Phase and coordination environment for dCu 2 O/Ag catalysts. a HAADF–STEM image with EDS elemental mappings and b high resolution STEM image of dCu 2 O/Ag 2.3%. c Enlarged XRD patterns for dCu 2 O, dCu 2 O/Ag 2.3% and dCu 2 O/Au 2.3% . d In situ XANES spectra and e Wavelet transform images of EXAFS data with optimized Morlet parameter (i.e., κ = 5, σ = 1) at Cu K-edge for commercial Cu-foil, dCu 2 O, dCu 2 O/Ag 2.3% and dCu 2 O/Au 2.3% . Fourier transform curves of in situ EXAFS data and corresponding fitted results (first coordination shell) for f dCu 2 O, g dCu 2 O/Ag 2.3% and h dCu 2 O/Au 2.3% . Scale bars, 10 nm in ( a ) and 1 nm in ( b ). Full size image To gain insight into the changed valence states and coordination environment of Cu following activation, operando X-ray absorption spectra (XAS) of Cu K-edge was recorded under activation conditions. The X-ray absorption near-edge structure (XANES) spectra show that the edge features for dCu 2 O, dCu 2 O/Ag 2.3% , and dCu 2 O/Au 2.3% are closed to those for the reference commercial Cu-foil. This finding confirms that the valence state for Cu for these catalysts decrease following activation to lie between 0 and +1, in following ordered sequence, dCu 2 O < dCu 2 O/Ag 2.3% < dCu 2 O/Au 2.3% (Fig. 2d ). The wavelet transform analysis confirms that the Cu–Cu region in all activated catalysts are located at ~6.7 Å −1 , suggesting that the alloyed CuAg and CuAu do not result in significant change in Cu–Cu bond length compared with the oxide-derived Cu (Fig. 2e ). The corresponding Fourier transform curves (from extended X-ray absorption fine structure (EXAFS) spectra) and fitted results of the first coordination shell for these activated catalysts show that the Cu–Cu coordination located at ~2.23 Å is the dominant structure in each sample, whilst there remains another Cu–O coordination peak at 1.35 Å for dCu 2 O/Ag 2.3% and dCu 2 O/Au 2.3%. This finding confirms that a significantly small fraction of Cu(I) remained for dCu 2 O/Ag 2.3% and dCu 2 O/Au 2.3% following activation (Fig. 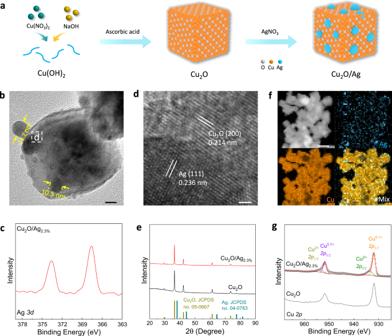Fig. 1: Structural characterization of Cu2O/Ag NCs. aSchematic for preparation of Cu2O/Ag NCs.bTEM image,cAg3dXPS curve,dHRTEM images andfEDS elemental mapping images of Cu2O/Ag2.3%NCs.eXRD patterns andgCu2pXPS curves for Cu2O and Cu2O/Ag2.3%NCs. Scale bars, 10 nm in (b), 1 nm in (d), and 100 nm in (f). White-color, orange and azure spheres in the model represent O, Cu, and Ag atoms, respectively. 2f–g and Supplementary Table 1 ). The coordination number for Cu−Cu in these catalysts was determined to equal, respectively, 11.4, 10.5, and 10.2 for dCu 2 O, dCu 2 O/Ag 2.3% , and dCu 2 O/Au 2.3% (Supplementary Fig. 9 ). Except for variation in Cu, the XPS for Ag 3d for dCu 2 O/Ag 2.3% shows that the binding energy for Ag 3d 5/2 shifts to a high level following activation. This evidences that the activation of alloying Ag with Cu induces electron transfer (Supplementary Fig. 10 ). Based on the foregoing, it is concluded that under electroreduction with highly significant structural rearrangement, the pristine metal-modified Cu 2 O NCs evolves to Cu-based bimetallics in a regulated valence and coordination environment. CO 2 RR performance CO 2 RR performance for the activated catalysts was directly evaluated via electrolyzing at specified currents (Supplementary Fig. 11 ). Figure 3a shows the linear sweep voltammetry curves for dCu 2 O, dCu 2 O/Ag 2.3% and dCu 2 O/Au 2.3% . 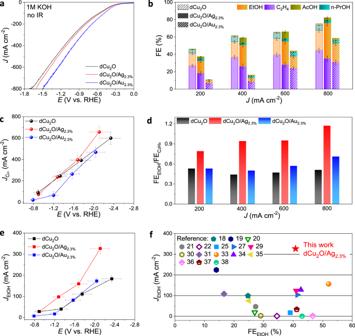Fig. 3: CO2RR performance for dCu2O, dCu2O/Au2.3%and dCu2O/Ag2.3%. aLinear sweep voltammetry curves toward CO2RR for dCu2O, dCu2O/Au2.3%and dCu2O/Ag2.3%.bFE value of C2+products for dCu2O, dCu2O/Au2.3%and dCu2O/Ag2.3%under selected current density.cPartial C2+current density andeC2+formationvspotential referred to reversible hydrogen electrode (RHE) on dCu2O, dCu2O/Au2.3%, and dCu2O/Ag2.3%.dRatio of FEEtOHto FEC2H4on dCu2O, dCu2O/Au2.3%, and dCu2O/Ag2.3%under selected current density.fEtOH partial current densityvsFEEtOHfor reported Cu-based catalysts. Error bars correspond to the standard deviation of three independent measurements. It is seen in the figure that the current density for CO 2 RR of dCu 2 O/Ag 2.3% and dCu 2 O/Au 2.3% are significantly increased, directly evidencing that modification boosted activity for CO 2 RR. The FEs were computed for liquid and gaseous product in the applied current range 200–800 mA in 1 M KOH by nuclear magnetic resonance (NMR, Supplementary Fig. 12 ) and gas chromatography (GC) (Supplementary Fig. 13 ) respectively. Figure 3b presents the FEs of C 2+ products (FEs C2+ ) for these catalysts under different current. C 2 H 4 and EtOH are the major C 2+ products, plus minor acetate and n–propanol. With the applied current increased, all catalysts exhibited increased FEs C2+ and a decreased FEs of CO (FEs CO ). Compared with the one–up FE C2+ for dCu 2 O from 200 to 400 mA, dCu 2 O/Ag 2.3% exhibits greater FE C2+ at significant current >  600 mA. Importantly, the total FE C2+ for dCu 2 O/Ag 2.3% is up to 82.1% at a current density 800 mA cm −2 , to exhibit the greatest partial C 2+ current density of 656.8 mA cm −2 and formation rate of 2042.2 μmol h −1 cm −2 at −2.11 V with reference to the reversible hydrogen electrode (V RHE , no iR correction, Fig. 3c and Supplementary Fig. 14a ). In contrast, the FE C2+ for dCu 2 O/Au 2.3% is significantly less than that for dCu 2 O/Ag 2.3% at all currents, confirming that the Au modification resulted in directly boosting only targeted CO generation, but not C–C coupling. Fig. 3: CO 2 RR performance for dCu 2 O, dCu 2 O/Au 2.3% and dCu 2 O/Ag 2.3% . a Linear sweep voltammetry curves toward CO 2 RR for dCu 2 O, dCu 2 O/Au 2.3% and dCu 2 O/Ag 2.3% . b FE value of C 2+ products for dCu 2 O, dCu 2 O/Au 2.3% and dCu 2 O/Ag 2.3% under selected current density. c Partial C 2+ current density and e C 2+ formation vs potential referred to reversible hydrogen electrode (RHE) on dCu 2 O, dCu 2 O/Au 2.3% , and dCu 2 O/Ag 2.3% . d Ratio of FE EtOH to FE C2H4 on dCu 2 O, dCu 2 O/Au 2.3% , and dCu 2 O/Ag 2.3% under selected current density. f EtOH partial current density vs FE EtOH for reported Cu-based catalysts. Error bars correspond to the standard deviation of three independent measurements. Full size image We analyzed the ratio of FE EtOH /FE C2H4 in C 2+ products at high current density on these catalysts. It is interesting that dCu 2 O/Ag 2.3% reaches the FE EtOH /FE C2H4 ratio 1.17 at an applied current 800 mA, which is significantly greater than that for dCu 2 O (0.51) and dCu 2 O/Au 2.3% of 0.71. This finding confirms that the Ag modification significantly inhibits C–O bond-breaking and stabilizes intermediates for EtOH vs C 2 H 4 (Fig. 3d ). Relying on the boosted FE EtOH of 40.8 % at a high current density (800 mA cm −2 ), the dCu 2 O/Ag 2.3% exhibits the greatest partial EtOH current density of 326.4 mA cm −2 at −2.11 V RHE (no iR correction, −0.89 V RHE with 85% iR correction, Supplementary Figs. 15 and 16 ). Importantly, this is 1.78 and 1.89 times greater than that for dCu 2 O and dCu 2 O/Au 2.3% , respectively (Fig. 3e ). The EtOH formation for dCu 2 O/Ag 2.3% could reach 1014.9 μmol h −1 cm −2 with current densities of 800 mA cm −2 at −2.11 V RHE (without iR correction) (Supplementary Fig. 14b ). 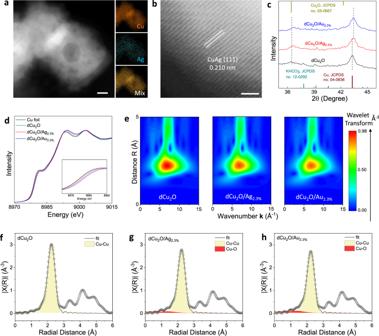Such highly significant performances for EtOH production on dCu 2 O/Ag 2.3% were compared directly with reported catalysts (Fig. Fig. 2: Phase and coordination environment for dCu2O/Ag catalysts. aHAADF–STEM image with EDS elemental mappings andbhigh resolution STEM image of dCu2O/Ag2.3%.cEnlarged XRD patterns for dCu2O, dCu2O/Ag2.3%and dCu2O/Au2.3%.dIn situ XANES spectra andeWavelet transform images of EXAFS data with optimized Morlet parameter (i.e.,κ= 5,σ= 1) at Cu K-edge for commercial Cu-foil, dCu2O, dCu2O/Ag2.3%and dCu2O/Au2.3%. Fourier transform curves of in situ EXAFS data and corresponding fitted results (first coordination shell) forfdCu2O,gdCu2O/Ag2.3%andhdCu2O/Au2.3%. Scale bars, 10 nm in (a) and 1 nm in (b). 3f , Supplementary Table 2 ). It is apparent that the dCu 2 O/Ag 2.3% exhibits the greatest reported partial EtOH current density amongst these, and represents the ‘best’ production for electroreduction of CO 2 to EtOH. In addition, the EE HC for EtOH on dCu 2 O/Ag 2.3% reaches 22.4% following iR correction under similar conditions, a value greater than that for most catalysts (Supplementary Fig. 16d ). In addition, the electrochemically active surface area (ECSA) for dCu 2 O/Ag 2.3% was computed via different methods and compared, together with mass normalized current density for EtOH (J ECSA (EtOH) and J mass (EtOH)) with independently reported studies (Supplementary Figs. 17 and 18 and Supplementary Table 3 ). The dCu 2 O/Ag 2.3% exhibited superior J ECSA (EtOH) and J mass (EtOH) compared with reported catalysts, confirming that the improved EtOH current density for dCu 2 O/Ag 2.3% is because of the intrinsic Ag-modified oxide-derived Cu sites and not the changed ECSA and mass loading of the catalyst itself. Based on these findings therefore of highly significant FE EtOH with high current density from dCu 2 O/Ag 2.3% on CO 2 RR, a series of Cu 2 O/Ag NCs with different amounts of modified Ag were assessed for CO 2 RR performance (Supplementary Figs. 19 and 20 ). Characterizations underscore that all pristine Cu 2 O/Ag NCs with different compositions exhibit similar structures, whereas the density of deposited NPs and oxidation state on the surface of Cu 2 O NCs increased with the degree of modification (Supplementary Fig. 21 ). From the comparison of the potential for CO 2 RR of different catalysts at a high current density of 800 mA cm −2 (Fig. 4a ), it can be seen that the demand potential decreases with increased Ag. This finding confirms the positive impact of Ag modification on CO 2 RR. The degree of introduced Ag-dependent FEs of products from these catalysts was assessed under the same current density. As is shown in Fig. 4b, c , increasing Ag in dCu 2 O/Ag leads to a volcano-shape for FE EtOH that corresponds with a reverse-volcano on FE CO , and contrasts with the monotonously decreased FE for C 2 H 4 . This correlation between the amount of modified Ag and FEs for CO and EtOH was observed also with other applied currents (Supplementary Fig. 22 ). Common to Cu-based catalysts, the coverage of CO on Cu surface is conducive to C–C coupling to impact EtOH and C 2 H 4 generation concurrently [24] . However, here for the dCu 2 O/Ag, only the FE for EtOH exhibits the dependent correlation with CO. These results indicate that the boosted EtOH is not only dependent on variable CO coverage on dCu 2 O/Ag, but also related to other unknown factors. Fig. 4: CO 2 RR performance for dCu 2 O/Ag with modified Ag. Comparison of a applied potentials, b FEs for C 1 and H 2 product, c FEs for C 2 H 4 and EtOH and total C 2+ product on dCu 2 O/Ag with modified Ag at current density 800 mA cm −2 . d Total current density and e FEs for C 2+ product for CO 2 RR on dCu 2 O/Ag 2.3% at selected cell voltage under MEA measurement. f Stability test for dCu 2 O/Ag 2.3% at the current density 800 mA cm −2 in MEA. Error bars correspond to the standard deviation of three independent measurements. Full size image The stability of dCu 2 O/Ag 2.3% was evaluated via long-term chronopotentiometry testing. It was found that there is no apparent decay of activity with 6 h continuous operation, in which the selectivity of EtOH decreased ~6% following CO 2 RR (Supplementary Fig. 23 ). TEM image and XRD pattern of spent dCu 2 O/Ag 2.3% showed that morphology and structure are maintained following the stability test (Supplementary Fig. 24 ). Given the superior EtOH production on dCu 2 O/Ag 2.3% , it was consequently assessed in a commercially relevant membrane electrode assembly (MEA) (Supplementary Fig. 25 ). It was found that there is a good, linear relationship between applied current and voltage in the MEA (Fig. 4e ). The FEs for all products tested in flow cell electrolyzer were well-reproduced in MEA (Supplementary Fig. 26 and Fig. 4d ), identifying that high current and high EtOH selectivity can be maintained under commercially relevant conditions (Fig. 4e ). Importantly, the durability of CO 2 RR in the catholyte–free MEA significantly outperformed the flow cell electrolyzer, which exhibited a decrease of FE EtOH (~3%) in 12 h operation under a full–cell voltage of −4.72 V with a total current density 800 mA cm −2 , evidencing the good stability of dCu 2 O/Ag 2.3% for CO 2 RR (Fig. 4f ). Mechanistic studies The CO reduction reaction (CORR) on dCu 2 O/Ag was assessed to identify whether boosted C–C coupling and EtOH generation followed a classic CO–tandem mechanism (Supplementary Fig. 27 ). To permit a direct comparison, the CORR behavior of dCu 2 O and dCu 2 O/Au 2.3% were evaluated and the catalysts were activated by a similar process with CO 2 RR. It was expected that if the CO–tandem mechanism dominated, the CORR performance for the catalysts would be similar [28] . However, as is shown in Supplementary Fig. 28 , the dCu 2 O/Ag 2.3% exhibits significant suppression of H 2 and promoted C–C coupling for C 2+ products under CORR. This is in significant contrast to dCu 2 O/Au 2.3% and dCu 2 O results. The partial current density of C 2+ products for dCu 2 O/Ag 2.3% reaches 696.0 mA cm −2 at –1.56 V RHE for CORR, and is significantly greater than those for dCu 2 O/Au 2.3% (~154.0 mA cm −2 ) and dCu 2 O (~188.0 mA cm −2 ). Similarly, the ratio FE EtOH /FE C2H4 for dCu 2 O/Ag 2.3% is also greater than that for dCu 2 O/Au 2.3% and dCu 2 O under CORR. Significantly, these findings from dCu 2 O/Ag 2.3% contrast with those for reported Cu–Ag catalyst with CO–tandem mechanism. This is interpreted that Ag modification results in intrinsic property changes in Cu active sites to: (1) suppress HER, (2) improve C–C coupling activity, and; (3) boost EtOH selectivity. In addition, the modification induced compressive strain, and morphology effects (crystal facets) for boosted EtOH production can be also excluded in our circumstances, because the exposed facets, surface structure and Cu–Cu bond length of both dCu 2 O/Au 2.3% and dCu 2 O/Ag 2.3% catalysts are similar. Therefore, other potential mechanisms on dCu 2 O/Ag 2.3% need to be assessed for boosted CO 2 RR performance. Reaction pathways for C 2 H 4 and EtOH production are similar on Cu surfaces, as they initiate with two adsorbed–CO dimerization followed by several steps of protonation and dehydration to generate a shared intermediate, * HCCOH [3] , [14] . The selectivity between C 2 H 4 and EtOH, is significantly dependent on the relative stabilities of the next-intermediates for EtOH and C 2 H 4 pathways branched from * HCCOH on Cu sites [3] , [14] , [40] . Cu with a relatively low coordinated surface and optimal oxide state is favorable for EtOH generation over C 2 H 4 because the reaction intermediates for EtOH are more saturated compared with those for C 2 H 4 [41] , and the existing oxidation is feasible to binding of key oxygen-bound intermediates for EtOH generation [33] , [42] . Combined with this and previous experiment results, it is hypothesized that Ag-induced the moderate coordinated surface and optimal oxidation of Cu in dCu 2 O/Ag 2.3% are responsible for boosted EtOH selectivity. Therefore, the CO 2 RR intermediates chemisorbed on dCu 2 O, dCu 2 O/Ag 2.3% , and dCu 2 O/Au 2.3% at different potentials were assessed via in situ attenuated total reflectance infrared absorption spectroscopy (ATR–IRAS) to determine the mechanism for boosted EtOH. As is shown in Fig. 5a, b and Supplementary Fig. 29 , with the cathode potential at −0.3 V RHE , the ATR–IRAS spectra for these catalysts exhibit several new peaks. 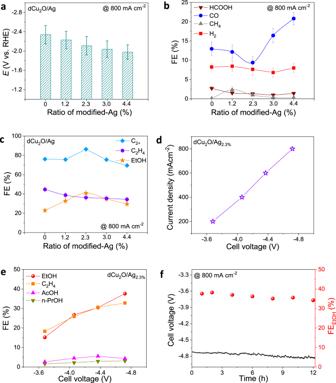Fig. 4: CO2RR performance for dCu2O/Ag with modified Ag. Comparison ofaapplied potentials,bFEs for C1and H2product,cFEs for C2H4and EtOH and total C2+product on dCu2O/Ag with modified Ag at current density 800 mA cm−2.dTotal current density andeFEs for C2+product for CO2RR on dCu2O/Ag2.3%at selected cell voltage under MEA measurement.fStability test for dCu2O/Ag2.3%at the current density 800 mA cm−2in MEA. Error bars correspond to the standard deviation of three independent measurements. These are assigned to corresponding intermediates based on independently reported studies (Supplementary Table 4 ). In particular, there appear two peaks at 2044 and 1923 cm −1 for dCu 2 O/Ag 2.3% , which are associated with the atop–adsorbed * CO ( * CO atop ) and bridge–adsorbed * CO ( * CO bridge ) on Cu surface, respectively [43] , [44] , [45] . In comparison, dCu 2 O and dCu 2 O/Au 2.3% mainly show the * CO atop peak with little evidence of * CO bridge binding in the same potential region. The different * CO binding configurations on these catalysts can also be observed from CO temperature-programmed desorption (CO–TPD) (Supplementary Fig. 30b ). Mathematical integration and statistical analyses confirm the ratio * CO bridge / * CO atop for dCu 2 O/Ag 2.3% is significantly greater than that for dCu 2 O or dCu 2 O/Au 2.3% over the potential range (Supplementary Fig. 31 and Fig. 5c ). These findings evidence that compared with dCu 2 O and dCu 2 O/Au 2.3% , the moderate coordination numbers and optimal oxidation for Cu surface in dCu 2 O/Ag 2.3% result in tailored * CO configuration. Given the different electron back-donating and proton-combining ability of adsorbed * CO on atop and bridge Cu sites, the energy barrier for following * CO protonation is altered. Previous studies demonstrate that * CO bridge protonation is more energetically favorable than that of * CO atop on Cu surface [46] . Therefore, the C–C coupling on dCu 2 O/Ag 2.3% could be triggered under asymmetry between * CO and * CHO (or * COH) following the * CO bridge protonation step. Notably, adsorbed * CHO intermediate was observed on dCu 2 O/Ag 2.3% from ATR-FTIR spectra, and increased with the applied potential (Fig. 5b ), strongly evidencing this process. This asymmetric C−C coupling has a lower energy barrier than that for *CO dimerization as evidenced by the reported theory studies [19] , which contributes to increased C 2+ production. Fig. 5: In situ ATR–IRAS measurement and mechanism for dCu 2 O/Ag 2.3% . In situ ATR–IRAS obtained during chronopotentiometry in a potential window 0.2 to −1.2 V RHE for a dCu 2 O, and b dCu 2 O/Ag 2.3% under CO 2 RR. (A reference spectrum obtained at 0.3 V RHE in 1 M KOH is subtracted). Potential dependence of ratio of c * CO bridge / * CO atop and d * OC 2 H 5 / * OCCOH obtained for dCu 2 O, dCu 2 O/Ag 2.3% and dCu 2 O/Au 2.3% . e Schematic for boosted EtOH generation over dCu 2 O/Ag 2.3% . Yellow-color, gray, white, orange, red, and azure spheres in the model represent H, C, O, Cu 1+ , Cu 0 , and Ag atoms, respectively. Full size image Additional peaks from ATR–IRAS spectra at ~1567 and ~1182 cm −1 and ~1336 and ~1117 cm −1 were analyzed. These peaks, indexed to the absorbed * OCCOH and * OC 2 H 5 on these catalysts, exhibit a ratio value for * OC 2 H 5 / * OCCOH on dCu 2 O/Ag 2.3% that is significantly greater compared with that for dCu 2 O and dCu 2 O/Au 2.3% . This finding evidences that the key * OC 2 H 5 intermediates for EtOH production are more stable on dCu 2 O/Ag 2.3% (Fig. 5d ) [42] , [43] . This is attributed to the asymmetric C−C coupling induced unbalanced coordination environment, which disrupts the coordination sites for C 2 H 4 intermediates, and thereby, stabilizes the EtOH intermediates. This is in agreement with report that diversity of * CO binding site enhances C 2+ liquid product formation [27] . Therefore we hypothesize that triggered asymmetric C−C coupling on dCu 2 O/Ag 2.3% boosts C 2+ production and favors EtOH pathway via stabilizing pivotal intermediates. In addition, the peak for the absorbed bicarbonate at 1547 cm −1 on dCu 2 O/Ag 2.3% is missing compared with dCu 2 O and dCu 2 O/Au 2.3% , confirming that the value of the local pH on the electrode of dCu 2 O/Ag 2.3% is greater than that for dCu 2 O and dCu 2 O/Au 2.3% during CO 2 RR [47] . The high pH at the surface of electrode is thought to favor C–C coupling by lowering the energy barrier of CO 2 activation and suppressing H 2 evolution, and contributes to the boosted activity for CO 2 RR. Moreover, the CO–TPD and CO 2 –TPD for dCu 2 O/Ag 2.3% also exhibit a higher temperature for CO 2 and CO desorption than those for dCu 2 O and dCu 2 O/Au 2.3 , indicating dCu 2 O/Ag 2.3% has stronger bonding strength of CO 2 and CO for efficient CO 2 RR at large current (Supplementary Fig. 30 ). Accordingly, based on the ATR–IRAS spectra analysis, the mechanism for boosted EtOH on dCu 2 O/Ag 2.3% can be soundly proposed (Fig. 5e ). At first, the coordinated pure-Cu surface is replaced with neighboring Ag atoms with modification by Ag in Cu 2 O and reduces these to CuAg alloy under CO 2 RR. Then, the Ag-induced moderate coordination numbers and optimal oxidation of Cu surface regulate binding strength of * CO, to configure mixed * CO bridge and * CO atop adsorption that triggers asymmetric C–C coupling after * CO bridge protonation. Because of the relatively low oxygen affinity and unsaturated nature of the C 2 H 4 intermediates compared with EtOH, the asymmetric C–C coupling provides an unbalanced coordination environment that is beneficial for EtOH intermediate formation and stabilization in lower energy than that for C 2 H 4 , and thereby promotes the pathway for EtOH. In summary, an assessment of a newly synthesized, silver-modified copper-oxide catalyst has confirmed that the CO 2 RR to EtOH pathway is accelerated via triggering the asymmetric C–C coupling. An optimized dCu 2 O/Ag 2.3% exhibits a FE of 40.8% and EE HF of 22.3% for EtOH production in flow cell, together with boosted EtOH partial current density of 326.4 mA cm −2 at −0.89 V RHE (with an 85 % iR correction). In situ ATR–IRAS spectroscopy confirmed that boosted EtOH selectivity results from moderate coordinated surface and optimal oxidation state of the Cu sites that gives mixed * CO bridge and * CO atop configurations for asymmetric C–C coupling to stabilize the EtOH intermediates. This demonstrated understanding of the mechanism for electroreduction of CO 2 –to– EtOH contrasts with reported, classic CO–tandem catalysis. It can be practically used to significantly boost EtOH production. Preparation of Cu 2 O, Cu 2 O/Ag, and Cu 2 O/Au NCs In a typical preparation for Cu 2 O/Ag 2.3% NCs, 0.5 mL NaOH solution (1 M) and 0.5 mL Cu(NO 3 ) 2 solution (0.1 M) were added to a 30 mL vial with 9 mL water under vigorous stirring for 5 min at RT to give a blue-color Cu(OH) 2 suspension. 27 mg AA was added to the vial under vigorous stirring. The suspension changed from blue color to yellow, confirming the formation of Cu 2 O NCs. Following stirring for 30 min, 0.1 mL AgNO 3 solution (0.01 M) was added to the vial, and stirring continued for 30 min. Cu 2 O/Ag 2.3% NCs were obtained and resulting products were collected by centrifugation and washed with EtOH. 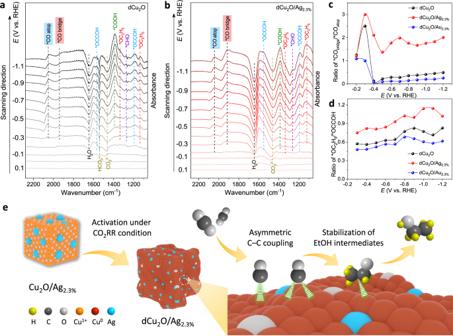Fig. 5: In situ ATR–IRAS measurement and mechanism for dCu2O/Ag2.3%. In situ ATR–IRAS obtained during chronopotentiometry in a potential window 0.2 to −1.2 VRHEforadCu2O, andbdCu2O/Ag2.3%under CO2RR. (A reference spectrum obtained at 0.3 VRHEin 1 M KOH is subtracted). Potential dependence of ratio ofc*CObridge/*COatopandd*OC2H5/*OCCOH obtained for dCu2O, dCu2O/Ag2.3%and dCu2O/Au2.3%.eSchematic for boosted EtOH generation over dCu2O/Ag2.3%. Yellow-color, gray, white, orange, red, and azure spheres in the model represent H, C, O, Cu1+, Cu0, and Ag atoms, respectively. Preparation of Cu 2 O and Cu 2 O/Au NCs was similarly conducted, but without the addition of AgNO 3 and with the replacement of AgNO 3 with HAuCl 4 •4H 2 O. Cu 2 O/Ag and Cu 2 O/Au NCs with different compositions were prepared by adding selected volumes of AgNO 3 and HAuCl 4 •4H 2 O solution (Supplementary Table 5 ). Characterizations TEM and HAADF–STEM were conducted on a FEI Tecnai F20 transmission electron microscope with an acceleration voltage 200 kV. Samples were prepared by dropping EtOH dispersions of the samples onto carbon-coated, Cu TEM grids using a pipette, and dried under ambient RT conditions. SEM images were taken with a HITACHI S–3700 cold–field emission scanning electron microscope operated at 15 kV. XRD patterns were collected on X’Pert–Pro MPD diffractometer (Netherlands PANalytical) with a Cu Kα X-ray source ( λ = 1.540598 Å). XPS was determined with an SSI S–Probe XPS Spectrometer. The carbon peak at 284.6 eV was used as a reference to correct for charging effects. XAS data were collected at the TPS–44 A beamline of the National Synchrotron Radiation Research Center (NSRRC, Hsinchu, Taiwan) using a Si (111) quick-scanning monochromator, and processed according to standard procedures using the Demeter program package (Version 0.9.24). CO 2 RR test in flow cell Electroreduction of CO 2 was tested in a microfluidics flow cell that consisted of two electrolyte chambers (20 × 5 × 3, mm) and one gas chamber (20 × 5 × 5, mm) [48] . An anion exchange membrane (Fumasep FAB–PK–130) was placed between two electrolyte chambers for products separation and ionic conduction. Catalyst-deposited GDE, micro Ag/AgCl electrode (4.0 M KCl), and Ni-foam (0.5 mm thickness), respectively, served as working electrode, reference electrode, and anode. To fabricate the working electrode, a certain amount of catalysts (3 mg) were dispersed in 1 mL EtOH with 20 µL 5 wt% Nafion solution and then sprayed onto a gas diffusion layer (CeTech, NIS1007) via airbrush. The loading amount of catalysts on GDE was controlled to ~0.44 mg cm −2 . The working electrode was placed between gas and catholyte chambers to ensure gaseous CO 2 diffusion and reaction at the catholyte/catalysts interface. The reference electrodes were inserted in catholyte chamber and maintained at a specified distance with the working electrode. An electrochemical workstation (CHI660, Chenhua, Shanghai) with a current amplifier was used to perform the CO 2 RR test. 1 M KOH (20 mL) was circulated through the electrolyte chambers under constant flow (15 mL min −1 ) via peristaltic pump. CO 2 was supplied into gas chambers by a mass-flow controller at a constant flow rate of 30 mL min −1 . Reactions were tested via chronopotentiometry at differing currents for 1 h without iR correction. Gas and liquid products were analyzed, respectively, via GC (Agilent 8890) and 1 H NMR (Agilent 600 MHz DirectDrive2 spectrometers). Potentials were referenced to RHE and iR correction performed based on the following, namely: 
    E_RHE=E_vs  Ag/AgCl+0.059 ×pH+ 0.210+0.85 × iR
 (1) where i is the current at each applied potential and R the equivalent series resistance measured via electrochemical impedance spectroscopy in the frequency. FE for the formation of CO 2 RR product was computed from: 
    FE=eF×n/Q=eF×n/(I×t)
 (2) in which e is the number of transferred electrons for each product, F the Faraday constant, Q charge, I applied current, t reaction time, and n total product (in mole). EE HC was computed on the basis of the cathodic CO 2 RR coupled with the anodic oxygen evolution reaction (O 2 + 4H + + 4e − ↔ 2H 2 O; 1.23 V vs RHE) from: 
    EE_HC=E_oe^∘ -E_red^∘/E_oe-E_red×FE_EtOH
 (3) where E oe o and E red o are, respectively, the thermodynamic potential for oxygen evolution and CO 2 RR to EtOH (0.08 V vs RHE), E oe and E red applied potentials at, respectively, anode and cathode. For the computation of the half-cell EE, the anodic reaction was assumed to occur with an overpotential of 0 V, that is, E oe = 1.23 V. CO 2 RR test in MEA Electroreduction of CO 2 in MEA consisted of two titanium backplates (TA2 grade) with a 4.0 cm 2 serpentine flow field, and MEA. Catalyst-deposited GDE (~0.44 mg cm −2 for Cu 2 O/Ag 2.3% NCs) and Ni-foam (0.5 mm thickness) were used, respectively, as cathode and anode. The cathode and anode were pressed onto sides of the anion exchange membrane (Sustainion 37–50, Dioxide Materials). The gap between the electrodes was minimized to reduce ohmic loss. Gaseous CO 2 (30 mL min −1 ) was passed behind the GDL to contact the catalyst, and 0.1 M solution was used as the anolyte which was circulated via pump at 20 mL min −1 . CO 2 RR performance for MEA was evaluated by applying different currents with a current amplifier in the two-electrode system at the CHI660 (Chenhua, Shanghai) electrochemical workstation. Cathodic gas products were vented through a simplified cold–trap to collect permeable liquid prior to gas chromatograph testing. FE values for the liquid products were computed based on the total mass of product collected on anode and cathode. ECSA measurement ECSA was measured by double-layer capacitance (DLC) and Pb underpotential deposition (Pb UPD) methods. All experiments are conducted in the flow cell and the used catalysts are obtained following activation under CO 2 RR. For DLC method, Cyclic Voltammetry (CV) scans were conducted at the potential range from 0.15 to 0.20 V vs RHE with increasing scan rates of 10, 20, 40, 60, 80, and 100 mV s −1 . The capacitance currents at 0.17 V vs RHE were plotted against the scan rates, and the double-layer capacitance (C dl , mF cm −2 ) was derived from the slope according to the following: 
    C_dl=I/v
 (4) where I is the capacitance current (half of the difference between the anodic current density and cathodic current density, (J a −J c )/2), and v is the scan rate. For Pb UPD method, the CV scans were conducted in Ar-saturated 0.01 M HClO 4 and 1 mM PbCl 2 at the potential range from 0.15 to 0.20 V vs RHE with scan rates of 10 mV s −1 . The ECSA of catalysts was determined according to the following: 
    ECSA_Pb UPD=A_Pb UPD/(320Ccm^-2v)
 (5) where A Pb UPD is the peak area of monolayer Pb stripping, v the scan rate and the constant 320 μC cm −2 is the charge density factor for the UPD of Pb on copper [33] . In situ ATR–IRAS measurement In situ ATR–IRAS was performed on a Nicolet iS20 spectrometer equipped with an HgCdTe (MCT) detector and a VeeMax III (PIKE Technologies) accessory. The measurement was conducted in a homemade electrochemical single-cell furnished with Pt–wire and Ag/AgCl as counter and reference electrodes. A fixed-angle Ge prism (60°) coated with catalysts embed into the bottom of the cell served as the working electrode. Before testing, the detector was cooled with liquid nitrogen for at least 30 min to maintain a stable signal. Chronoamperometry was used for CO 2 RR test and was accompanied by the spectrum collection (32 scans, 4 cm −1 resolution). All spectra were subtracted with the background.